Large Rashba spin splitting of a metallic surface-state band on a semiconductor surface The generation of spin-polarized electrons at room temperature is an essential step in developing semiconductor spintronic applications. To this end, we studied the electronic states of a Ge(111) surface, covered with a lead monolayer at a fractional coverage of 4/3, by angle-resolved photoelectron spectroscopy (ARPES), spin-resolved ARPES and first-principles electronic structure calculation. We demonstrate that a metallic surface-state band with a dominant Pb 6 p character exhibits a large Rashba spin splitting of 200 meV and an effective mass of 0.028 m e at the Fermi level. This finding provides a material basis for the novel field of spin transport/accumulation on semiconductor surfaces. Charge density analysis of the surface state indicated that large spin splitting was induced by asymmetric charge distribution in close proximity to the nuclei of Pb atoms. One of the challenges in developing semiconductor spintronics is to generate spin-polarized electrons at room temperature [1] , [2] . A partial solution is spin injection from ferromagnets, which has seen significant progress for GaAs [3] . Although semiconductor devices are also proposed for spin filtering [4] and generation of spin-polarized current [5] , [6] on the basis of the Rashba spin splitting [7] , [8] for two-dimensional electrons, these have not yet been realized. Recently, the Rashba effect at crystal surfaces [9] , [10] has been discovered to exhibit spin splitting orders of magnitude larger than those at semiconductor heterojunctions, and sometimes comparable with the separation between conduction bands [11] , [12] . For a spintronic application of the surface giant Rashba effect, (i) a large spin splitting of (ii) a metallic surface-state band on (iii) a semiconductor surface is required. The first and second requisites are because of the requirement for significant spin transport, and the third is indispensable because the large bulk current in metallic substrates sweeps off any surface spin signals. In this paper, we show that a large Rashba spin splitting is realized for a metallic surface-state band on a semiconductor surface. This opens a new field of surface spin transport/accumulation [13] , which also has implications for efficient spin accumulation, filtering and injection into semiconductors. The surface Rashba effect was first discovered on Au(111) [9] , [10] and then on other metal surfaces such as W [14] , Bi [15] and Bi-covered Ag [11] , [12] . The charge density distribution along the surface normal in the vicinity of the nuclei is crucial for the surface Rashba effect because the potential gradient is most prominent at closest proximity to nuclei [16] . Premper et al . [17] suggested that the size of Rashba spin splitting could be further enhanced by the existence of in-plane structural inversion asymmetry. The studies on Bi/Ag systems indicated that large Rashba spin splitting is possible even on the surface of a light element when it is covered with a monolayer of a heavier element. This accelerated the search for the large Rashba effect on semiconductor surfaces such as Si and Ge, as this has potential importance in spintronic applications. Although some studies have been carried out on the Rashba effect on heavy-element-covered Si(111) and Ge(111) surfaces [18] , [19] , [20] , [21] , [22] , [23] , [24] , these studies show only nonmetallic spin-split bands, which contribute little to spin transport, or lack direct experimental evidence of spin splitting. Pb thin films with a thickness of ∼ 10 monolayers on Si(111) were shown to exhibit a Rashba spin-split quantum-well state [25] . The films, however, had a high density of spin-degenerated metallic bands and hence would not exhibit detectable spin-dependent transport properties. Thus, it is of crucial importance to establish a semiconductor surface with Rashba spin-split metallic surface bands. In this paper, we report on the Rashba spin splitting of a metallic surface-state band on a Ge(111) surface induced by a Pb monolayer. 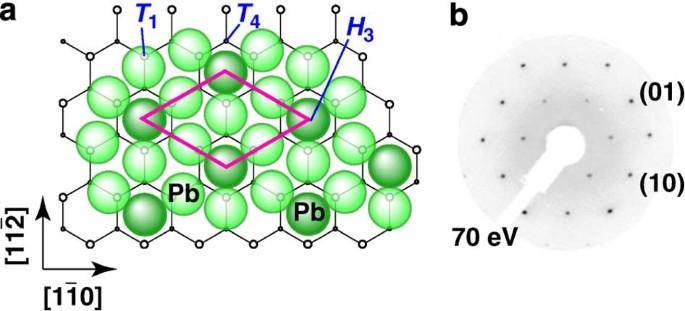Figure 1: Schematic structure model and low-energy electron diffraction (LEED) pattern of Pb/Ge(111). (a) Top view of. The large and small circles indicate Pb adatoms and Ge atoms in the first bilayer, respectively. The solid parallelogram denotes the unit cell. (b) LEED pattern of. Angle-resolved and spin-resolved photoelectron spectroscopy Figure 1a shows the structural model [26] and low-energy electron diffraction pattern of the surface. The nominal Pb coverage is 4/3, with one of four Pb atoms per unit cell located at an H 3 site and the other three on off-centred bridge positions between T 1 and T 4 sites. Figure 1: Schematic structure model and low-energy electron diffraction (LEED) pattern of Pb/Ge(111). ( a ) Top view of . The large and small circles indicate Pb adatoms and Ge atoms in the first bilayer, respectively. The solid parallelogram denotes the unit cell. ( b ) LEED pattern of . 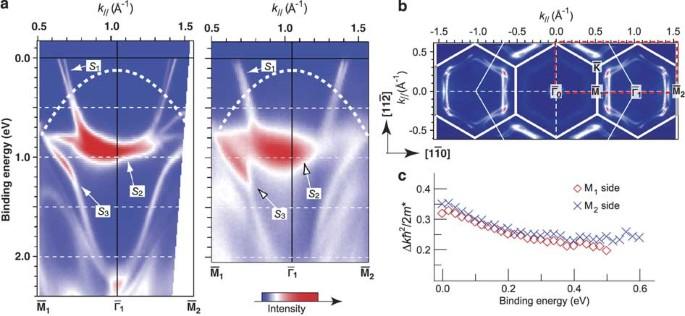Figure 2: Energy band dispersion measured by ARPES. (a) Experimental energy band dispersions along112of thesurface Brillouin zone (SBZ) at 30 K and room temperature are shown in the left and right panels, respectively. The dashed line indicates the upper edge of the projected bulk bands of Ge(111). (b) Fermi surface map. The bold dashed (red) rectangle shows the region actually measured. The rest of the image was obtained by mirror symmetry operations. Bold and thin solid lines denoteand (1×1) SBZs, respectively. (c) Momentum splitting Δk||, multiplied by2/2m*, forS1in theM1(diamonds) andM2(crosses) sides as a function of binding energy. Full size image Figure 2a shows the band dispersion along 1 1 2 measured by angle-resolved photoelectron spectroscopy (ARPES) at 30 K (left panel) and at room temperature (right panel). Three Pb-induced bands denoted as S 1 , S 2 and S 3 can be clearly seen. These bands are not observed on the clean Ge(111)-c(2×8) surface. The S 1 band, which is located in the projected bulk band gap and crosses the Fermi level, E F , is clearly split into two. Although the bands are thermally broadened at room temperature, the S 1 band clearly shows splitting near E F . At binding energies greater than ∼ 0.4 eV, the S 1 band is merged into the projected bulk bands. The effective mass for the S 1 band is estimated to be 0.028 m e at E F . Figure 2b was obtained by imaging the photoelectron intensity within a 50 meV energy window centred at E F and it shows the Fermi surface due to S 1 . The Fermi surface is composed of two concentric hexagons, which agrees with expectations for the Rashba spin-split bands. Figure 2: Energy band dispersion measured by ARPES. ( a ) Experimental energy band dispersions along 1 1 2 of the surface Brillouin zone (SBZ) at 30 K and room temperature are shown in the left and right panels, respectively. The dashed line indicates the upper edge of the projected bulk bands of Ge(111). ( b ) Fermi surface map. The bold dashed (red) rectangle shows the region actually measured. The rest of the image was obtained by mirror symmetry operations. Bold and thin solid lines denote and (1×1) SBZs, respectively. ( c ) Momentum splitting Δ k || , multiplied by 2 /2 m *, for S 1 in the M 1 (diamonds) and M 2 (crosses) sides as a function of binding energy. 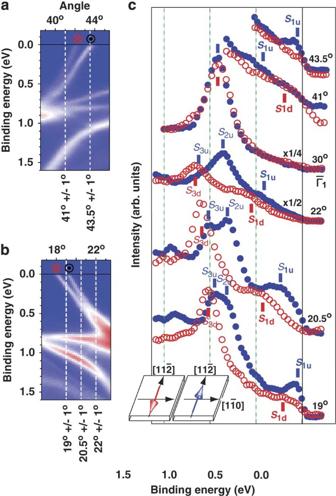Figure 3: Spin-resolved ARPES. (a,b) Spin-unpolarized ARPES. Dashed lines indicate the angles for which spin-resolved ARPES are shown. (c) Spin-resolved ARPES spectra measured at several selected angles along112. The probed spin orientation axis is parallel to, which is parallel to the surface and perpendicular to. The intensities for spin-up and spin-down, defined as spins oriented towardsand, respectively, are plotted by the blue solid and red open circles, respectively. Full size image Figure 3c shows spin-resolved ARPES spectra taken at several selected angles along 1 1 2 in the direction. Energy and angular resolution were set at 110 meV and 2.0°, respectively. It was found that the spectra for spin-up and spin-down measured at the emission angle of 30° are almost identical and show the S 2 peak at ∼ 0.9 eV. The emission angle of 30° corresponds to the 1 point. This indicates that the spin-up and spin-down states of S 2 are degenerate at , as expected for the Rashba splitting. The good overall agreement of the spin-up and spin-down spectra indicates the high accuracy of the present spin-resolved measurement. Figure 3: Spin-resolved ARPES. ( a , b ) Spin-unpolarized ARPES. Dashed lines indicate the angles for which spin-resolved ARPES are shown. ( c ) Spin-resolved ARPES spectra measured at several selected angles along 1 1 2 . The probed spin orientation axis is parallel to , which is parallel to the surface and perpendicular to . The intensities for spin-up and spin-down, defined as spins oriented towards and , respectively, are plotted by the blue solid and red open circles, respectively. Full size image Except for the spectra taken at 30°, the spectra for spin-up and spin-down show k || - and binding-energy-dependent asymmetry. In particular, the S 1 and S 3 states show clear energy splitting, depending on the spin polarization. For emission angles of 19°, 20.5° and 22° ( 1 side), the spin-up peaks of S 1 and S 3 are located at lower binding energies than the corresponding spin-down peaks. Comparing the spin-unpolarized ARPES data, we find that the higher (lower) binding energy branch of the S 1 band is spin-down (spin-up). For emission angles of 41° and 43.5° ( 2 side), the positions of the spin-up and spin-down branches of the S 1 band are inverted; that is, the spin-up branch is located at binding energies higher than the spin-down branch. Note that the spin-down branch is above E F for emission angle 43.5°. These results indicate that the splitting observed by ARPES for the S 1 band is due to Rashba spin splitting. The spin polarization for the S 1 band at emission angles of 22° and 41° may be small because the band is merged into the projected bulk bands. On the other hand, although the S 3 band does not appear to be split in the spin-unpolarized spectra, spin-resolved data suggest that S 3 is also spin-split up to ∼ 100 meV. The binding energy dependence of the momentum splitting Δ k || for S 1 times 2 /2 m * is plotted in Fig. 2c . The Δ k || values were evaluated by fitting the momentum distribution curves with two Gaussian functions. Note that the ideal Rashba model for two-dimensional free electrons yields two free-electron-like parabolas that are shifted in opposite k || directions by a constant value from the point. The Rashba parameter is then expressed by the momentum splitting Δ k || as α R =Δ k || 2 /2 m *. The observed momentum splitting for S 1 shows an almost constant value, Δ k || =0.028±0.002 Å −1 , in the binding energy range of 0.2–0.6 eV. The Rashba parameter is therefore deduced to be α R =0.24±0.02 eV Å −1 . On the other hand, momentum splitting in the binding energy range of 0–0.2 eV deviates from the constant value and reaches Δ k || =0.04 Å −1 at E F . The energy splitting value between the spin-up and spin-down states for S 1 is 200 meV at k F1 =0.36 Å −1 . 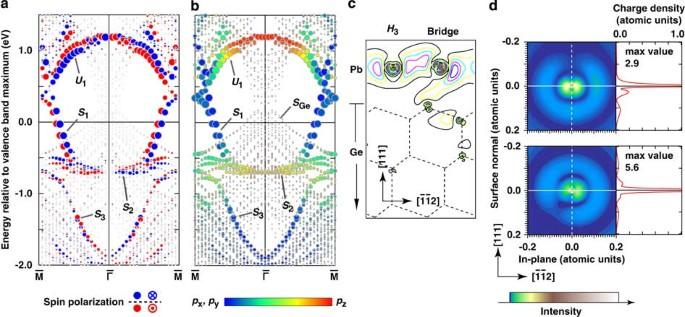Figure 4: Calculated band structure and charge density distribution. (a) Band structure calculated for thesurface. The spin quantization axis is. Opposite spin orientations are indicated by blue and red circles. The radii of the blue (red) circles are proportional to the net contribution of Pb 6pwith spin-up (spin-down). (b) Band structure with relative contributions of Pb 6pxpyand 6pzshown by colour scale. The sizes of the circles are proportional to the total contribution of Pb 6p. (c) Charge density contour for the state at whichS1crossesEF. (d) (Top panel) Charge density distribution near a Pb nucleus located at theH3site (left) and line profile along the surface normal (dashed line) (right);z=0 corresponds to the nuclear position. (Bottom panel) The same as the upper panel but for Pb located at the bridge site. First-principles calculation Figure 4a,b shows the calculated band structure. The spin quantization axis is , which is perpendicular to k || ( 1 ). In Fig. 4a , the radii of the circles are proportional to the net contribution of Pb 6 p , with the spin oriented towards (blue) and (red), indicating spin splitting of the Pb-induced bands. The U 1 , S 2 and S 3 bands are in resonance with the bulk bands near , which prevents unambiguous identification of a Rashba-type k || -linear spin splitting near . However, the absence of spin polarization at , as indicated by the absence of circles in Fig. 4a , is consistent with Rashba-type spin splitting. In Fig. 4b , the radii of the circles are proportional to the total contribution of Pb 6 p , and the colour index represents the relative contributions of Pb 6 p x p y and 6 p z . The calculation reproduces the characteristic Pb-induced features, S 1 , S 2 and S 3 , observed by ARPES. The S 1 band has a strong Pb 6 p x p y character. The S 3 band also has a Pb 6 p x p y character and a larger contribution from Ge orbitals. The S 2 and unfilled U 1 bands have characters of bonding and antibonding, respectively, between Pb 6 p z and Ge 4 p z of the topmost Ge atoms. Figure 4: Calculated band structure and charge density distribution. ( a ) Band structure calculated for the surface. The spin quantization axis is . Opposite spin orientations are indicated by blue and red circles. The radii of the blue (red) circles are proportional to the net contribution of Pb 6 p with spin-up (spin-down). ( b ) Band structure with relative contributions of Pb 6 p x p y and 6 p z shown by colour scale. The sizes of the circles are proportional to the total contribution of Pb 6 p . ( c ) Charge density contour for the state at which S 1 crosses E F . ( d ) (Top panel) Charge density distribution near a Pb nucleus located at the H 3 site (left) and line profile along the surface normal (dashed line) (right); z =0 corresponds to the nuclear position. (Bottom panel) The same as the upper panel but for Pb located at the bridge site. Full size image The calculation indicates that the split pairs of S 1 are spin polarized in opposite directions, in agreement with the result of spin-resolved ARPES. Spin splitting is calculated to be 165 meV at k F1 =0.366 Å −1 , in good agreement with the experiment. The dispersion calculated for S 2 and S 3 bands is also in agreement with the ARPES and spin-resolved ARPES. Thus, we conclude that the experimentally observed splitting is due to the Rashba effect. We also note that the Ge-derived surface state ( S Ge ) appears just above the bulk bands in the vicinity of the point. This state has negligible contribution from Pb orbitals. The size of the Rashba splitting for the S 1 band is orders of magnitude larger than that of semiconductor quantum wells (typically a few meV). Simulations of spin-dependent phenomena such as spin accumulation/transport and spin filtering for Rashba spin-split surface bands have been reported recently [27] , [28] , [29] . It should, however, be difficult to study the spin transport phenomena experimentally on the previously known metallic-surface Rashba systems, because these are all based on metallic substrates, and large bulk current interferes as background. The Pb/Ge(111) system now serves as an ideal prototype for surface spin transport. Several types of nonequilibrium spin-dependent transport/accumulation phenomena are expected to be observed, as the surface conductivity on this surface should be dominated by the electrons in the spin-split S 1 band. An experiment along this line is underway. The charge density contour for the S 1 state at E F is shown in Fig. 4c , which indicates that the state is mostly localized in the Pb monolayer. The contributions of different Pb atomic orbitals to the wavefunction of the S 1 state are in the ratio 6 s :6 p =1:5.5. The 6 p component is predominantly of in-plane character as shown in Fig. 4b . According to Nagano et al . [16] , the size of Rashba spin splitting is determined by the integral of the potential gradient along the surface normal times the charge density, Because the potential gradient is most prominent at closest proximity to the nuclei, the charge density asymmetry along z in the vicinity of the nuclei governs the splitting. The charge density profiles in the z direction near the Pb nuclei are illustrated in Fig. 4d . Whereas for Pb at the bridge position, the distribution shows a nearly symmetric feature near z =0, the Pb atom on the H 3 site exhibits an asymmetric charge distribution at | z |<0.05 a.u. (atomic units: 1 a.u.=0.529 Å), which therefore makes a dominant contribution to the Rashba spin splitting. In principle, the Rashba spin splitting at surfaces can be as large as the spin-orbit splitting in a free atom [16] , as for Bi/Ag [11] , [12] . The spin splitting observed here is considerably smaller than the spin-orbit splitting of the 6 p orbital in a free Pb atom, 1.75 eV, which is because the S 1 band is predominantly of an in-plane p character. A larger contribution of s and p z , which could be possible for different adsorption geometry, would lead to more prominent charge density asymmetry along the z direction and hence to a larger spin splitting. We conclude that a metallic surface-state band on Pb/Ge(111) exhibits a Rashba spin splitting of 200 meV and an effective mass of 0.028 m e at E F , thus serving as a basis for surface spin transport. The size of the spin splitting is larger by a factor of 8 than the thermal energy k B T at room temperature. The low effective mass is important because it is associated with a high electron mobility. As the effect does not depend on any peculiar properties of Ge, it would be possible to realize a similar electronic structure on a Si surface. Once a spin asymmetry is induced on the Si surface, whether by spin filter, spin accumulation or any other effect, it enables spin injection into the substrate. It is also possible to grow a thin epitaxial Ge film on a Si substrate and then deposit Pb on it to obtain surface spin asymmetry. In addition, the surface would be covered by a stable insulating film such as metal oxide without destroying the surface electronic state, which enables us to study various properties under ambient conditions. Sample preparation method The ARPES experiment was performed in an ultrahigh-vacuum system with a base pressure of 1.0×10 −10 Torr. A Ge(111) substrate was prepared by several cycles of 0.7 keV Ar + bombardment and subsequent annealing up to 870 K for a few seconds. Pb was deposited onto the surface at room temperature, which was then annealed at 570 K for 10 min. ARPES and spin-resolved ARPES The intensities of the low-energy electron diffraction pattern ( Fig. 1b ) and the Pb 5 d photoemission were monitored to optimize the Pb coverage. ARPES measurements were carried out by a hemispherical electron energy analyser (VG Scienta R3000) in an angular mode and monochromatized He I α radiation ( hν =21.218 eV). The sample was maintained at 30 K or at room temperature during the ARPES measurement. The spin-resolved ARPES experiments were performed at Hiroshima Synchrotron Radiation Center (HSRC), Hiroshima University, using He I α radiation and a Mott detector operating at 25 keV [30] , [31] . In the spin-resolved ARPES measurement, the sample temperature was kept at 100 K. First-principles calculation First-principles calculation was performed using the WIEN2K computer code on the basis of the 'augmented plane wave+local orbitals' (APW+lo) method [32] with the spin-orbit interaction being taken into account. The surface was modelled by repeated slabs consisting of a 24-layer Ge(111) slab, with one side covered with a layer and the opposite side terminated by hydrogen atoms. Starting from the structural model determined by X-ray diffraction, [26] the atomic positions were optimized until the root mean square of the forces exerted on all the atoms becomes negligibly small (<2 mRy per a.u. ). How to cite this article: Yaji, K. et al . Large Rashba spin splitting of a metallic surface-state band on a semiconductor surface. Nat. Commun. 1:17 doi: 10.1038/ncomms1016 (2010).